Evidence for activity-regulated hormone-binding cooperativity across glycoprotein hormone receptor homomers Glycoprotein hormone receptors show strong negative cooperativity. As a consequence, at physiological hormone concentrations, a single agonist binds to a receptor dimer. Here we present evidence that constitutively active receptors lose cooperative allosteric regulation in direct relation with their basal activity. The most constitutive mutants lost nearly all cooperativity and showed an increase of initial tracer binding, reflecting the ability of each protomer to bind with equal affinity. Allosteric interaction between the protomers takes place at the transmembrane domain. The allosteric message resulting from hormone binding to the ectodomain of one protomer travels 'downward' to its transmembrane domain, before affecting the transmembrane domain of the other protomer. This results in transmission of an 'upward' message lowering the binding affinity of the ectodomain of the second protomer. Our results demonstrate a direct relation between the conformational changes associated with activation of the transmembrane domain and the allosteric behaviour of glycoprotein hormone receptors dimers. G protein-coupled receptors (GPCRs), the largest family of membrane proteins, are integral parts of interaction networks, which have crucial roles in cellular homeostasis [1] . Glycoprotein hormone receptors (GpHrs) constitute a subfamily of rhodopsin-like GPCRs responsible for signal transduction by thyrotropin (TSH), lutropin or chorionic gonadotropin (LH/CG), and follitropin (FSH) [2] , [3] . Because cells express several GPCR subtypes, signal transduction is both temporally and spatially integrated to generate the appropriate cellular response on activation of several receptors. Over the past years, the concept of GPCR homo- or hetero-oligomerization has generally been accepted [4] , and GpHrs are no exception [5] , [6] . GpHrs show a division of labour between agonist binding, by a large ectodomain (ECD) made of leucine-rich repeats, and G protein (mainly Gαs) activation, by a canonical rhodopsin-like transmembrane domain (TMD). Whereas direct structural information is only available for the leucine-rich repeat portion of the ECD of the follicle-stimulating hormone receptor (FSHr) and thyroid-stimulating hormone receptor (TSHr) [7] , [8] , access to the structure of ligand-free [9] , agonist- [10] , inverse agonist- [11] or antagonist-bound [12] , constitutively active mutant [13] and G protein-bound [14] class A GPCR crystals has deepened our understanding of the conformational rearrangement involved in activation of the serpentine portion of GpHrs. In agreement with their bi-partite structure, activation of GpHrs deviates from the mechanisms implicated in the activation of the majority of class A GPCRs devoid of large ECDs. Whereas direct interaction between the agonist and different regions of the TMD takes place for the majority of GPCRs, a favoured current model holds that GpHr activation involves switching of the ECD from an inverse agonist into a tethered agonist of the TMD, on binding of the hormone [3] , [15] . This model provides a rational explanation to the observation that the TSHr can be activated by binding of ligands with little, if any sequence identity (TSH, thyrostimulin, autoantibodies) as well as by point mutation in a specific residue of the ECD [3] , [16] , [17] . A large number of activating mutations (CAMs) have been identified in GpHrs that may be responsible for a variety of endocrine phenotypes [17] . Interestingly, although most of these are located in the rhodopsin-like TMD, in the case of the FSHr, they allosterically impact on hormone specificity [18] , [19] . The mechanisms or structures that regulate the reciprocal interaction between the ECD and TMD are unclear at the present time. They likely involve the 'hinge' region connecting ECD to TMD, the structure of which remains unknown. Increasing evidence points to a connection between GPCR homo(hetero)meric complexes and ligand-binding cooperativity [20] , [21] , [22] although caution is needed [23] , [24] . Concerning GpHr homomers, we and others have demonstrated that negative cooperativity regulates high affinity hormone binding. Ligand binding to one of the protomers decreases the binding affinity of the other protomer, so that a single agonist molecule would bind a receptor homomer under physiological (low) hormone concentrations [25] , [26] . Such inter-protomeric communication might allow sensitive regulation of the target cell by low hormone concentrations, while showing effective but less sensitive responses to high ligand concentrations [27] . Importantly, we were able to demonstrate that, at least for TSHr, this allosteric regulation is present in a native system, where the receptor is expressed at its normal level and in its physiological environment. The possibility to make a GPCR homomer function with a single ligand molecule has been documented in other systems [28] , [29] . With the aim of exploring the allosteric communication between the partners of a GPCR homomer, we investigated the effect of artificially activating the receptors on their binding characteristics. Using the 'infinite dilution' method [30] , [31] as a read-out of the cooperative interaction, we demonstrate an inverse relation between constitutive activity and negative cooperativity in all the three GpHrs tested. Our data provide evidence to support a model in which the TMD tunes the affinity and selectivity of the interaction between the hormone and the ECD. Constitutively active TSHr mutants and cooperativity Whereas the existence of higher order oligomers is highly probable [32] and is actually supported by the present data, we will use the words dimer and homo-oligomer interchangeably and, for simplicity, we will attempt to model the behaviours of homodimers only. To investigate how the protomers communicate within a GpHr homomer, we evaluated the effect of ligand-independent constitutive activity on TSHr hormone binding. To avoid direct influence of mutations on the binding site, thereby introducing potential structural bias, we explored several point mutations known to be constitutively active [33] , [34] , [35] and randomly distributed in the receptor sequence ( Fig. 1a , color corresponds to each substitution). Indeed, as reported before, all these point mutations caused an increase in basal cyclic AMP accumulation that, when normalized to the level of expression of each mutant allows sorting them according to their 'specific constitutive activity' [35] ( Fig. 1b ). We next performed radioligand homologous (same tracer and unlabelled competitor) binding competition experiments and noted that, with few exceptions, the constitutively active mutants show a significant enhancement of the initial specific binding (Bo) with little or no change in the IC 50 ( Fig. 1c ). The increase in Bo was not due to a greater mutant receptor surface level of expression when compared with wild type (WT) ( Fig. 1d ). Actually, when Bo are normalized to cell surface expression, all the constitutively active receptors show higher values than the WT receptor ( Fig. 1e ). Interestingly, with the exception of S281L mutant, the normalized Bo show a direct saturable relation with the level of constitutive activity ( Fig. 1f ). It is likely that the outlier behaviour of S281L reflects the location of the substituted residue in the ECD, which may affect its binding properties. 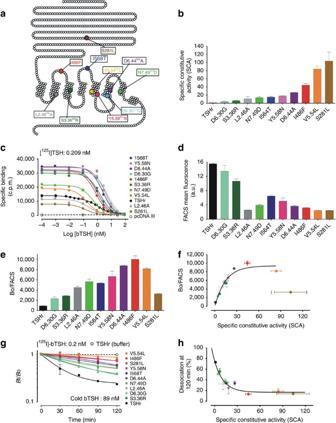Figure 1: Constitutively active TSHr mutants and negative cooperativity. (a) Cartoon representing the location of the selected constitutively active TSHr mutants. Mutant receptors are colour-coded and numbered according to the Ballesteros and Weinstein nomenclature59for the substitutions located in the TM and following Swiss-Prot for the extracellular (ECD and ECL) mutations. (b) Constitutive cAMP accumulation normalized as explained in Methods, (c) radiolabelled TSH homologous competition binding, (d) and surface expression by FACS using monoclonal anti-TSHr BA8 were quantified in COS-7 cells transiently expressing WT or constitutively active TSHr. (e) Normalization of initial binding (Bo) over cell surface expression (f) correlates with constitutive activity. (g) A large excess (89 nM) bTSH induced acceleration of 0.2 nM [125I]-bTSH was measured in the same cells as explained in Methods. (h) 120 min dissociation against the normalized constitutive activity. Spearman's coefficient: −0.89,P-value two-tailed=0.0005. Representative experiments are shown out of at least three independent experiments performed with duplicate samples. Data are presented as Mean±s.e.m. and binding competition (c) or exponential decay (g,h) nonlinear regression was used to fit the corresponding experimental observation. Figure 1: Constitutively active TSHr mutants and negative cooperativity. ( a ) Cartoon representing the location of the selected constitutively active TSHr mutants. Mutant receptors are colour-coded and numbered according to the Ballesteros and Weinstein nomenclature [59] for the substitutions located in the TM and following Swiss-Prot for the extracellular (ECD and ECL) mutations. ( b ) Constitutive cAMP accumulation normalized as explained in Methods, ( c ) radiolabelled TSH homologous competition binding, ( d ) and surface expression by FACS using monoclonal anti-TSHr BA8 were quantified in COS-7 cells transiently expressing WT or constitutively active TSHr. ( e ) Normalization of initial binding (Bo) over cell surface expression ( f ) correlates with constitutive activity. ( g ) A large excess (89 nM) bTSH induced acceleration of 0.2 nM [ 125 I]-bTSH was measured in the same cells as explained in Methods. ( h ) 120 min dissociation against the normalized constitutive activity. Spearman's coefficient: −0.89, P -value two-tailed=0.0005. Representative experiments are shown out of at least three independent experiments performed with duplicate samples. Data are presented as Mean±s.e.m. and binding competition ( c ) or exponential decay ( g , h ) nonlinear regression was used to fit the corresponding experimental observation. Full size image As shown previously [26] , [36] , [37] , the rate of dissociation of radiolabelled TSH from the WT receptor is strongly accelerated in the presence of a large excess of cold hormone ( Fig. 1g , black symbols), and this behaviour has been shown to reflect negative cooperativity of TSHr homomers [26] . When tested under the same conditions, all mutant receptors showed a decrease in the rate of tracer dissociation compared with WT ( Fig. 1g ; Supplementary Fig. S1a , SF S1a). Interestingly, a negative correlation was observed between the level of constitutive activity and the acceleration of tracer dissociation, suggesting that negative cooperativity is inversely related to basal receptor activity ( Fig. 1h ). On the basis of our assumption that negative cooperativity results from allosteric interactions between receptor protomers in a dimer or oligomer [26] , the observed reduction in allosteric behaviour of the mutants could be due to reduction of their ability to dimerize. Homogeneous time resolve fluorescence resonance energy transfer (HTRF) experiments demonstrated that constitutively active receptors are able to homomerize similarly to the WT receptor ( Supplementary Fig. S1b ) in the expression range we have studied. The observed difference in the slopes of the curves in Supplementary Fig. S1b likely reflects differences in the geometry of the complexes, because they show no relation with specific constitutive activity of the mutants (the strongest mutant tested, V5.54L, behaves as the WT). We accordingly exclude a reduction in molecular proximity as the cause of the reduced allosteric regulation of the hormone binding. Alternatively, the decrease in tracer dissociation observed for the mutants could conceivably be secondary to increased internalization of constitutively active receptors, shielding them from the cell surface more prominently than the WT on agonist binding. We could exclude this possibility because a similar inverse relation between constitutivity and dissociation kinetics was observed in membrane preparations from transiently transfected cells ( Supplementary Fig. S1c , inset). As the mutant receptors were all expressed at lower levels than the WT ( Fig. 1d ), we performed radioligand dissociation experiments in cells transfected so that they show surface expression ( Supplementary Fig. S2c,d ) or Bo ( Supplementary Fig. S2a,b ) similar to the WT receptor. In both cases, a strong inverse correlation was observed between the basal activity and the negative binding cooperativity ( Supplementary Fig. S2b,d; insets). Together with the observation of a direct saturable relation between Bo and specific constitutive activity of mutants ( Fig. 1f ), this excludes that the observed loss of allosteric behaviour of the mutants would result from a trend towards 'absolute negative cooperativity'. In this case, indeed, the most constitutively active mutants would be expected to show lower, rather than higher Bo (a single tracer per monomer, at most). On these bases, we conclude that negative binding cooperativity is genuinely altered in the constitutively active receptors. Enhanced basal activity changes binding stoichiometry Inspection of TSH binding curves on Fig. 1c reveals that many mutants show an increase in Bo, despite lower expression at the cell surface ( Fig. 1d ). When normalized to the expression level, even those with a lower absolute Bo (L2.46A, S281L) show increased binding on a molar basis ( Fig. 1e ). As the IC 50 of the mutants and the WT are similar ( Fig. 1c ), the higher Bo is not due to increased binding affinity, which again suggests that the mutations tend to decrease negative cooperativity. The observation that normalized binding of TSH to the most constitutive mutants is higher than twice that of the WT (the theoretical maximum for a dimer without negative cooperativity) suggests that we may be dealing higher order homomers, rather than simply dimers [32] . We then proceeded to determine the binding affinity K d1 , reflecting interaction of a single hormone molecule with the homomer, and K d2 that would reflect the affinity of the higher order homomer, when it is already occupied by one ligand. For this, we needed to determine association ( k on ) and dissociation ( k off ) constants for both sites ( K d1 = k off1 / k on1 ; K d2 = k off2 / k on2 ). The k on2 , k off1 and k off2 could be determined from the radioligand dissociation kinetics in the absence or the presence of increasing concentrations of unlabelled TSH ( Fig. 2a–d ) and from the curves displaying evolution of the k obs as a function of ligand concentrations ( Fig. 2e ) ( Supplementary Notes 1 and 2 ). However, in the case of receptors showing extreme reduction in ligand-induced dissociation (like I486F), the calculation of the k on2 becomes very challenging because of the reduced dynamic range for the effect. Therefore, K d2 could not be determined accurately for such receptors. We then quantified k on1 by following the rate of tracer association over time ( Fig. 2f ). The results of these computations are summarized in Table 1 and show an inverse relation between constitutive activity and k off2 , with no significant changes in K d1 , ultimately resulting in a reduction of the ratio between the affinities of both sites (α= K d2 / K d1 ). In agreement with the comparison of the initial binding values described above (Bo, Fig. 1c ) we conclude that the WT TSHr binds to a single hormone per homomer with high affinity at concentrations around the K d1 , whereas the most constitutively active receptors may bind multiple hormones per homomer. 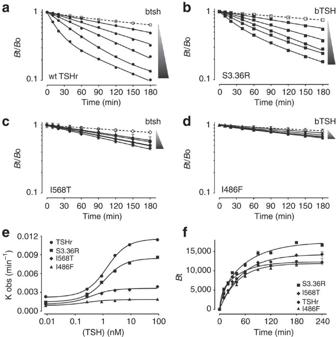Figure 2: Constitutive activity modifies second low affinity binding site. (a–d) Dissociation of prebound 0.2 nM [125I]-bTSH in the presence of buffer or increasing concentrations of bTSH was quantified in COS-7 cells transiently expressing WT or a subset of constitutively active TSHr mutants. The triangle represents the extent of the dissociated tracer. (e) Representing k obs, obtained from the dissociation profile shown ina–d,over the bTSH used to chase the tracer, and according to the mathematical model explained inSupplementary Notes 1 and 2,we calculated both sites' dissociation constants (koff1andkoff2) and the second site's association constant (kon2). (f) Association binding experiments performed with 0.2 nM [125I]-bTSH over 4 h allowed elucidation ofkon1fromkobsas perkon1=(kobs−koff)/L*. These parameters are summarized inTable 1. Representative experiments are shown out of two independent experiments with duplicate samples. Data are presented as Mean±s.e.m. and exponential decay (a–d), sigmoidal dose response (e) or exponential association (f) nonlinear regression was used to fit the corresponding experimental observation. Figure 2: Constitutive activity modifies second low affinity binding site. ( a – d ) Dissociation of prebound 0.2 nM [ 125 I]-bTSH in the presence of buffer or increasing concentrations of bTSH was quantified in COS-7 cells transiently expressing WT or a subset of constitutively active TSHr mutants. The triangle represents the extent of the dissociated tracer. ( e ) Representing k obs, obtained from the dissociation profile shown in a – d ,over the bTSH used to chase the tracer, and according to the mathematical model explained in Supplementary Notes 1 and 2, we calculated both sites' dissociation constants ( k off1 and k off2 ) and the second site's association constant ( k on2 ). ( f ) Association binding experiments performed with 0.2 nM [ 125 I]-bTSH over 4 h allowed elucidation of k on1 from k obs as per k on1 =( k obs − k off )/L*. These parameters are summarized in Table 1 . Representative experiments are shown out of two independent experiments with duplicate samples. Data are presented as Mean±s.e.m. and exponential decay ( a – d ), sigmoidal dose response ( e ) or exponential association ( f ) nonlinear regression was used to fit the corresponding experimental observation. Full size image Table 1 Summary of the dissociation and association kinetic parameters for WT or constitutively active TSHr. Full size table To confirm that reduction of the negative cooperativity accompanying the increase in constitutive activity might cause a change in the ligand:homomer stoichiometry, we took advantage of chimeric receptors harbouring a WT TSHr TMD and either the FSHr (FT) or the hCG/LHr (LT) ECD [38] . Coexpression of an excess of the chimeric FT ( Fig. 3a ) with either WT or I486F TSHr did not modify the surface expression of TSHr ( Fig. 3a ). It resulted, however, in a significant enhancement of the [ 125 I]-bTSH Bo only for the WT TSHr ( Fig. 3b ). We interpret these results in the following way: on titration of TSHr homomers with FT, the TSHr–FT heteromers are expected to lose regulation by a second cooperative site as FT does not bind TSH [38] . The result is an increase in Bo ( Fig. 3b ) despite comparable surface expression of WT TSHr ( Fig. 3a ). In a similar experiment performed with the I486F mutant, no increase in initial binding was observed when it was coexpressed with the FT chimera ( Fig. 3b ), suggesting that I486F homomer was able to bind more than one TSH molecule when expressed alone. Moreover, when we repeated the titration experiments by coexpressing a large excess of the LT chimera with either WT TSHr or the I486F mutant ( Fig. 3c ), we were able to measure a high-affinity hCG 'competition' component to [ 125 I]-bTSH binding only in cells coexpressing LT and the WT TSHr ( Fig. 3d ), but not the I486F mutant. We verified that the I486F-LT heteromer was present at the plasma membrane ( Fig. 3d, inset) excluding a loss of molecular proximity as the cause of the lack of hCG competition. This supports the idea that TSH binding is preserved at the constitutive protomer, and negative cooperativity is not transmitted when one TMD is constitutively active. Together, these experiments confirm that constitutively active receptor homomers show an increase in ligand binding stoichiometry. 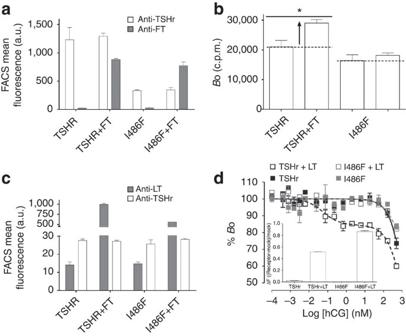Figure 3: Constitutively active receptors bind more than one agonist molecule per homomer. We measured surface receptor expression (a,c), radioligand binding (b,d) and HTRF (dinset) in whole HEK 293T cells transiently expressing WT or constitutive I486F mutant receptor alone or together with a large excess of chimeric receptors composed by either FSHr (FT) (a,b) or LH/CGr ECD (LT) (c,d) and a WT TSHr TMD. (a,c): Surface TSHr was quantified using anti-TSHr BA8, FT using anti-FSHr 5B2 and LT using anti-LH/CGr 16B5 monoclonal antibodies and anti-mouse-FITC as secondary as explained in Methods. (b) Initial binding (Bo) was quantified after incubating 0.2 nM [125I]-bTSH 4 h, and statistical significance was evaluated by a non-parametric unpaired two tailedt-test (*P=0.0171). (d) 0.2 nM [125I]-bTSH and increasing concentrations of hCG were incubated for 4 h and a two-site competition was only detected for cells coexpressing WT TSHr and LT (IC50for the first site=0.037±0.017 nM, fraction: 15.20%). (d, inset) HTRF was performed by incubating the cells expressing different receptor combinations with 16B5-cryptate (anti-LH/CGr) as the donor with anti-TSHr Iri-Sab2-AF647 as the acceptor for 1 h at 37 °C, and energy transfer was quantified as explained in Methods. Representative experiments are shown out of three independent experiments with duplicate samples. Data are presented as Mean±s.e.m. and one- or two-site competition binding (d) nonlinear regression was used to fit the corresponding experimental observation. Figure 3: Constitutively active receptors bind more than one agonist molecule per homomer. We measured surface receptor expression ( a , c ), radioligand binding ( b , d ) and HTRF ( d inset) in whole HEK 293T cells transiently expressing WT or constitutive I486F mutant receptor alone or together with a large excess of chimeric receptors composed by either FSHr (FT) ( a , b ) or LH/CGr ECD (LT) ( c , d ) and a WT TSHr TMD. ( a , c ): Surface TSHr was quantified using anti-TSHr BA8, FT using anti-FSHr 5B2 and LT using anti-LH/CGr 16B5 monoclonal antibodies and anti-mouse-FITC as secondary as explained in Methods. ( b ) Initial binding (Bo) was quantified after incubating 0.2 nM [ 125 I]-bTSH 4 h, and statistical significance was evaluated by a non-parametric unpaired two tailed t -test (* P =0.0171). ( d ) 0.2 nM [ 125 I]-bTSH and increasing concentrations of hCG were incubated for 4 h and a two-site competition was only detected for cells coexpressing WT TSHr and LT (IC 50 for the first site=0.037±0.017 nM, fraction: 15.20%). ( d , inset) HTRF was performed by incubating the cells expressing different receptor combinations with 16B5-cryptate (anti-LH/CGr) as the donor with anti-TSHr Iri-Sab2-AF647 as the acceptor for 1 h at 37 °C, and energy transfer was quantified as explained in Methods. Representative experiments are shown out of three independent experiments with duplicate samples. Data are presented as Mean±s.e.m. and one- or two-site competition binding ( d ) nonlinear regression was used to fit the corresponding experimental observation. Full size image Activity-caused cooperativity reduction is a general signature When we first reported the link between receptor dimerization and negative binding cooperativity the phenomenon was observed in all three GpHrs [26] . To determine whether the relationship between negative cooperativity and hormone-independent basal activity is a general characteristic of this particular class A GPCR subfamily, we studied the allosteric behaviour of a panel of constitutively active FSHr and LH/CGr mutants ( Fig. 4a,c ). Of note, whereas FSHr constitutively active mutations are located in the TMD ( Fig. 4a ) and are associated with promiscuous hormone selectivity [5] , [18] , [19] , [39] , the residues we tested in constitutive LH/CGrs are located in the ECD or extracellular loops (ECL) ( Fig. 4c ). As for the TSHr, there was an inverse correlation between the degree of constitutive activity and the extent of the ligand-accelerated tracer dissociation for both receptors ( Fig. 4b,d ). Also, similar to the results with TSHr mutants, an increase in Bo, relative to the WT, was observed in binding experiments performed with the clinically relevant [19] , [40] D6.30G FSHr mutant ( Fig. 4e ), despite slightly lower expression ( Fig. 4f ). In addition, the competition binding curve of the WT FSHr was best fit by assuming a two-site binding model, whereas a single-site fit was sufficient to account for competition of FSH binding to the D6.30G mutant ( Fig. 4e ). We conclude that constitutive activation in the three studied GpHrs alters negative cooperativity and homomer:ligand stoichiometry in a similar manner. 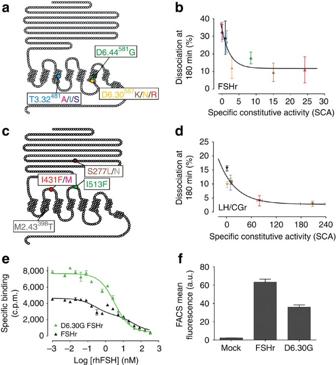Figure 4: Constitutively active receptors behave similarly in other GpHrs. Cartoon representation recapitulating the studied substitutions in both FSHr (a) and LH/CGr (c) that serves also as colour code. 0.4 nM [125I]-hFSH (b) and 0.9 nM [125I]-hLH (d) dissociation kinetics in the absence or presence of a large excess of the unlabelled agonist (330 nM rhFSH and 163 nM hCG) were performed and measured as explained forFig. 1and in Methods in COS-7 transiently expressing WT or different constitutively active FSHr or LH/CGr. Constitutive cAMP accumulation was performed and quantified exactly as explained in Methods. Representation of the percentage of dissociation at 180 min against the specific constitutive activity (SCA) reveals a negative correlation between negative cooperativity and constitutive activity. (e) 0.4 nM [125I]-hFSH binding was competed with increasing concentrations of rhFSH in COS-7 cells transiently expressing WT or D6.30G FSHr. (f) Surface expression of WT and constitutive FSHr evaluated by FACS. Representative experiments are shown out of three independent experiments with triplicate samples. Data are presented as Mean±s.e.m. and exponential decay (b,d) or one-or two-site competition binding nonlinear regression (e) was used to fit the corresponding experimental observation. Spearman's coefficient −0.95 andP-value=0.0011 for FSHr (b) and −0.90 andP-value=0.03 for LH/CGr (d). Figure 4: Constitutively active receptors behave similarly in other GpHrs. Cartoon representation recapitulating the studied substitutions in both FSHr ( a ) and LH/CGr ( c ) that serves also as colour code. 0.4 nM [ 125 I]-hFSH ( b ) and 0.9 nM [ 125 I]-hLH ( d ) dissociation kinetics in the absence or presence of a large excess of the unlabelled agonist (330 nM rhFSH and 163 nM hCG) were performed and measured as explained for Fig. 1 and in Methods in COS-7 transiently expressing WT or different constitutively active FSHr or LH/CGr. Constitutive cAMP accumulation was performed and quantified exactly as explained in Methods. Representation of the percentage of dissociation at 180 min against the specific constitutive activity (SCA) reveals a negative correlation between negative cooperativity and constitutive activity. ( e ) 0.4 nM [ 125 I]-hFSH binding was competed with increasing concentrations of rhFSH in COS-7 cells transiently expressing WT or D6.30G FSHr. ( f ) Surface expression of WT and constitutive FSHr evaluated by FACS. Representative experiments are shown out of three independent experiments with triplicate samples. Data are presented as Mean±s.e.m. and exponential decay ( b , d ) or one-or two-site competition binding nonlinear regression ( e ) was used to fit the corresponding experimental observation. Spearman's coefficient −0.95 and P -value=0.0011 for FSHr ( b ) and −0.90 and P -value=0.03 for LH/CGr ( d ). Full size image Structural determinants that support the information flow TSHr is one of the most constitutively active GPCR. In contrast, the human FSHr is almost silent in the absence of agonist in our expression system ( Supplementary Fig. S3 ). As constitutive activity seemed related to a decrease in the cooperative regulation between the two protomers in a homomeric complex, we reasoned that determining the accelerated dissociation rate in a chimeric FT (with TMD and ECD coming from a 'noisy' TSHr- and 'silent' FSHr-receptor, respectively) could be useful for identifying the part of the receptor implicated in the transmission of the allosteric signal. As shown in Fig. 5a , when we followed FSH dissociation kinetics in FT-expressing cells, we observed a spontaneous (non-excess ligand induced) dissociation that greatly resembled the TSHr-[ 125 I]-bTSH off-rate (TSHr–TSH results are shown as reference). Interestingly, [ 125 I]-hFSH dissociation was less marked for the FT when compared with WT FSHr, suggesting that introduction of a constitutive TMD decreased the negative cooperativity, reminiscent of the data obtained with the single-point mutations in all three receptors. 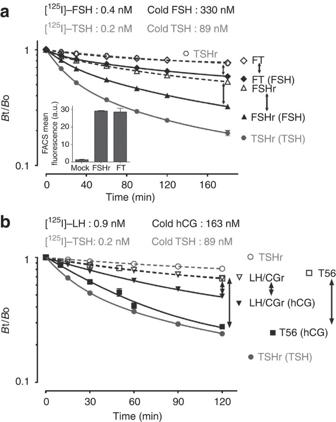Figure 5: The TMD is crucial for negative binding cooperativity across the dimer. 0.4 nM [125I]-hFSH (a) and 0.9 nM [125I]-hLH (b) dissociation kinetics in the absence (open symbols and dashed lines) or presence (filled symbols and continuous lines) of a large excess of the unlabelled agonist (330 nM rhFSH and 163 nM hCG) were performed and measured as explained forFig. 1and in Methods in COS-7 transiently expressing WT or different chimeric receptors. TSHr dissociation kinetics are shown in grey as reference, and the arrows represent the extent of each dissociation profile to allow direct comparison between WT or chimeric receptors when the same radioligand and excess were used. (a, inset) Surface WT or chimeric FSHr expression evaluated with 5B2. Representative experiments are shown out of three independent experiments with triplicate samples. Data are presented as Mean±s.e.m., and exponential decay nonlinear regression was used to fit the corresponding experimental observation. Figure 5: The TMD is crucial for negative binding cooperativity across the dimer. 0.4 nM [ 125 I]-hFSH ( a ) and 0.9 nM [ 125 I]-hLH ( b ) dissociation kinetics in the absence (open symbols and dashed lines) or presence (filled symbols and continuous lines) of a large excess of the unlabelled agonist (330 nM rhFSH and 163 nM hCG) were performed and measured as explained for Fig. 1 and in Methods in COS-7 transiently expressing WT or different chimeric receptors. TSHr dissociation kinetics are shown in grey as reference, and the arrows represent the extent of each dissociation profile to allow direct comparison between WT or chimeric receptors when the same radioligand and excess were used. ( a , inset) Surface WT or chimeric FSHr expression evaluated with 5B2. Representative experiments are shown out of three independent experiments with triplicate samples. Data are presented as Mean±s.e.m., and exponential decay nonlinear regression was used to fit the corresponding experimental observation. Full size image Finally, we further explored the nature of the structural determinant involved in inter-protomeric communication, using a TSHr construct capable of binding TSH and hCG with equally high affinity [41] . This mutant (T56) contains a WT TSHr TMD and an ECD with dual binding characteristics [26] , [41] . If, apart from being the minimal unit necessary for receptor homomerization [26] , the TMD is also the scaffold implicated in transmitting the allosteric signal, acceleration of dissociation of [ 125 I]-LH from the T56 mutant should resemble dissociation of [ 125 I]-bTSH from the WT TSHr, and be different from dissociation of [ 125 I]-LH from WT LH/CGr. As shown in Fig. 5b , this is exactly what is observed. Together, these experiments point to the TMD as the effector of the allosteric communication and show that the allosteric regulation is independent of the nature of the hormone, because LH dissociates very efficiently from the ECD of a receptor construct that contains a TSHr TMD. We have previously reported a direct functional link between GpHr di(oligo)merization and negative cooperative behaviour [26] : hormone binding to one protomer within the homomer decreases the affinity of the other(s), so that, at physiological hormone concentrations, a single ligand molecule binds to a receptor homomer. This effect is particularly marked in the TSHr, but is definitely present in the FSHr and LH/CGr [26] as well. Negative cooperativity introduces asymmetry in the ligand-bound receptor dimer at the binding level, raising the question whether it also causes asymmetrical activation of each protomer. This is of particular interest in GpHrs in which ligand binding and activation of G protein capability take place in specialized domains (the ectodomain, ECD- and transmembrane domain, TMD-, respectively). With the aim of exploring the allosteric communication between protomers (horizontal communication among protomers) or domains (vertical communication in the same protomer), we investigated how imposing symmetry at the transmembrane level by artificially activating the receptors would affect their binding characteristics. Our results show that mutants rendered constitutively active by amino-acid substitutions affecting the TMD, the ECLs or the hinge between the ECD and the TMD, lose negative cooperativity in direct relation to their level of basal activity ( Figs 1 and 4 ). In other words, forcing symmetry at the TMD level, by enhancing the population of protomers in the active state, translates into symmetry at the ligand-binding level, allowing binding with high affinity of one hormone molecule to each protomer of the homomer. A detailed analysis of the binding kinetics shows that it is the k off (dissociation rate) of the second site that is decreased in constitutive mutants ( Fig. 2 and Table 1 ). It must be stressed that in the model used to compute the kinetic parameters ( Supplementary Notes ), only dimers have been considered, meaning that K d2 reflects the affinity of the homomer when it is already occupied by one ligand. Also, the possible asymmetry introduced by binding of a single G protein per activated homomer has not been considered. Di(oligo)merization of GPCRs is reportedly mediated by interactions between transmembrane helices [32] , [42] , [43] . For GpHrs, both TMD-alone and ECD-alone constructs have been shown to dimerize efficiently [7] , [26] . Allosteric communication could thus theoretically take place at both levels. However, our results with chimeric receptors composed of the constitutively active TSHr TMD and the ECD from the silent FSHr point to the TMD as the site of allosteric communication between protomers responsible for negative cooperativity ( Figs 3a and 5a ). This is compatible with recent data demonstrating that GPI-anchored TSHr ECD lose their allosteric behaviour [25] , and provides a plausible explanation for the observation that crystals of the FSHr ECD show dimers with two molecules of FSH bound [7] . Asymmetric agonist binding to WT GPCRs is compatible with the current notion that assumes that activation of one GPCR protomer is not only sufficient, but may favour signal transduction within a GPCR complex [28] , [29] , [44] . Indeed, binding of an agonist to one protomer is able to activate a dopamine D2 receptor homomeric complex, and binding of an inverse agonism to the second site enhances signalling [28] . However, as reported by Han et al . [28] , this asymmetry is not only observed with ligand-induced conformational selection but also beyond ligand-binding cooperativity, because agonist-independent activation in a constitutive receptor is enough to propagate an inhibitory effect to the partner receptor and decrease the efficacy of the homomeric complex. A clear case of an asymmetric binding mode has been dissected in chemokine receptor homo- and hetero-mers (reviewed in ref. 45 ). Such allosteric behaviour is also responsible for the gain of opioid receptor function observed when treating a chemokine-opioid receptor heteromer with a chemokine receptor antagonist [46] . These considerations extend beyond the field of chemokine receptors and may be patho-physiologically important [47] , [48] . However, asymmetry may not be a general requirement for maximal activation of GPCRs, as there are clearly cases in which binding of an agonist to each member of a homomer activates more efficiently G protein coupling [49] . In one particular case, it has been suggested that binding of one TSH molecule to the high-affinity site of a dimeric TSHr would activate Gαs, while binding of a second would allow activation of both Gαs and Gαq [50] . This provides an elegant rationale for the observed dual coupling of human TSHr, with activation of Gαq requiring higher hormone concentrations [51] . In GPCRs in which the agonist binds directly to the TMD, the effect of ligand-dependent or mutation-induced activation of one protomer on the functional or binding characteristics of the dimer may essentially be viewed as reflecting 'horizontal' allosteric communication between protomers. In GpHrs, the situation is more complex as there is a clear division of labour between binding (to the ECD) and signalling (by TMD). The normal mode of activation of GpHrs by a hormone implies intramolecular 'top-down' vertical communication between the ECD and the TMD. Substantial experimental evidences indicate that an intermediary domain linking the ECD to the TMD, the 'hinge' domain, has a crucial role in this communication: (i) mutation of a serine residue, highly conserved in the hinge domain of all three GpHrs, activates the receptor constitutively [52] , [53] ; (ii) sulfation of tyrosine residues present in the hinge is required for efficient activation of all three receptors by their cognate hormone [54] ; (iii) the hinge region harbours an epitope which, when recognized by a monoclonal antibody, dramatically decreases the basal activity of the WT or constitutively active mutants [55] . The existence of a reciprocal, 'bottom-up', communication between the TMD and the ECD is evident in the mutant FSHr present in patients with ovarian hyperstimulation syndrome [19] , [40] , [56] . The majority of these mutants show various degree of constitutive activity secondary to amino-acid substitutions in the TMD and show promiscuous activation by both chorionic gonadotropin and TSH [39] . In addition, these constitutively active hFSHr can be activated by hCG unlike the WT hFSHr [19] , [40] , [56] . This loss of selectivity of the FSHr resulting from increased basal activity is a property not shared by either TSHr [39] or LH/CGr [57] . These observations suggest that, although not directly involved in hormone binding, the TMD has a critical role in the selectivity of activation by glycoprotein hormones. In addition, the present results indicate that the TMD also controls the stoichiometry of hormone binding to the ECDs of a homomer and provide new information on 'bottom-up' communication from TMD to ECD. Indeed, a chimeric receptor made of the FSHr ECD upstream of the TSHr TMD shows a decrease of negative cooperativity, compared with the WT FSHr ( Fig. 5a ). That the TSHr TMD confers TSHr-like constitutive activity to the chimera is reminiscent of the inverse relation between constitutive activity and negative cooperativity observed in TSHr mutants ( Fig. 1f ). The bottom-up communication between the TMD and the ECD seems to depend essentially on the nature of the TMD, as a mutant TSHr with amino-acid substitutions in the ECD allowing it to bind TSH and hCG with the same affinity, shows TSHr-like allosteric behaviour ( Fig. 5b ). The results described here point to a model of allosteric behaviour of GpHrs homomers in which 'horizontal' communication between the TMDs is implicated in an asymmetric mode of activation. In this respect, GpHrs behave similarly to many classical rhodopsin-like GPCRs devoid of an ECD. However, the modular structure of GpHrs, with distinct domains involved in binding and signalling, confers an important role on the hinge region connecting 'vertically' the ECD and TMD. On hormone binding to the ECD of one protomer, the hinge region would transduce 'downwards' the activation signal to its cognate TMD. This would result in asymmetric activation of the homomer and propagation of an inactivating signal horizontally to the other TMDs of the homomer. The hinge region would in turn convey an 'upwards' signal to the unbound ECDs, resulting in the observed negative binding cooperativity. Forcing activation of TMDs within the homomer, as in constitutively active mutants, would impose symmetrical conformation at the ECD level, thus erasing the cooperative behaviour. Reagents Plasmid pcDNA 3.1 from Invitrogen (Merelbeke, Belgium); plasmid pSVL from Amersham Pharmacia Biotech (Roosendaal, The Netherlands); restriction enzymes from Life Technologies (Merelbeke, Belgium) and New England Biolabs (Beverly, MA, USA). mAb BA8, Iri-Sab2, 16B5 and 5B2, obtained by classical genetic immunization [58] , are directed against different epitopes on the TSHr (BA8 and Iri-Sab2), LH/CGr and FSHr ECDs, respectively; OR2-15A-6 (mAb Anti-RT (rho-tagged)) was kindly provided by P. Hargrave (Department of Ophthalmology, University of Florida, Gainesville, FL, USA). Recombinant hCG and purified bovine (b) TSH were from Sigma Chemical (St Louis, MO, USA) or from BRAHMS Diagnostics (Berlin, Germany); recombinant human (rh) FSH from Organon Belge (Brussels, Belgium); [ 125 I]-bTSH was from BRAHMS and [ 125 I]-hLH and [ 125 I]-hFSH were labelled in-house. Ultrapure pituitary hLH and hFSH were obtained from the National Program of Hormone Production (Harbor-UCLA, LA). Receptor constructs All the constructions were engineered by subcloning available mutant receptors. TSHr mutations were created by subcloning the mutant receptors already constructed in pSVL [33] , [35] into the Afl III /Xba I or Bsu 36I /Xba I-digested pcDNA3.1-SPRT-TSHr cDNA. For LH/CGr, the previously constructed mutant receptors (Rodien and Bonomi, unpublished) were subcloned into the Hin dIII /Bam HI-digested pcDNA3.1-SPRT-LH/CGr cDNA. Finally, the FSHr mutants were also subcloned from existing mutant receptors [39] by subcloning into the Eco RV /Xba I-digested pcDNA3.1-SPRT-FSHr cDNA. All constructs were sequenced for mutation confirmation. Transfection experiments COS-7 cells were cultured, expressed and used as previously described [41] for all the cAMP determinations, most of the FACS and the radioligand binding experiments, whereas HEK 293T cells used for HTRF, a subset of the radioligand-binding experiments and the accompanying FACS experiments. Cell surface expression Expression of WT, chimeric and mutant receptors (RT or not) was quantified by FACS with the mAb BA8 (anti-TSHr), 16B5 (anti-LH/CGr), 5B2 (anti-FSHr) or the mAb OR2-15A-6 (anti-RT) exactly as explained previously [58] . Determination of cAMP production cAMP determinations were performed as previously described [41] . Duplicate samples were assayed in all experiments; results are expressed in pmol ml −1 . Concentration-effect curves were fitted with Prism v5.0 and EC 50 calculated. Specific constitutive activity was calculated exactly as described previously [35] , based on the linear relationship existing between basal cAMP accumulation and receptor surface expression. Binding assays Ligand binding was measured on either COS-7 or HEK 293T cells expressing either WT, chimeric or mutant receptors. The experiments were done and analysed exactly as previously published for both radioligand competition and dissociation kinetics experiments [26] . For some of the experiments ( Figs 2 and 5 ), we introduced a sequential binding whereby we removed and quantified the radioactivity of the supernatant at each point. The total specific radioactivity was the product of the sum of all the different amounts of radioactivity at each time point. We previously evaluated that the method show comparative results as the reference method. Antibody labelling for HTRF The monoclonal antibodies were labelled in-house with the maleimide derivative of the europium cryptate (diMP) (donor) and Alexa Fluor 647 (AF647) (Molecular Probes) as acceptor, as described previously [26] . HTRF measurements HEK 293T cells expressing increasing amounts of the wild-type or mutant receptors were collected, resuspended in PBS and distributed in a black 96-well reading plate (VWR) where 0.5 μg ml −1 donor-labelled antibody and 5 μg ml −1 acceptor labelled antibody were already present. After 1 h, at 37 °C, readings were performed and FRET signal are represented as Delta F (ΔF). Cells transfected with the empty vector or expressing other receptor were always used as negative controls. How to cite this article: Zoenen, M. et al . Evidence for activity-regulated hormone-binding cooperativity across glycoprotein hormone receptor homomers. Nat. Commun. 3:1007 doi: 10.1038/ncomms1991 (2012).